Platelet production proceeds independently of the intrinsic and extrinsic apoptosis pathways BH3 mimetic drugs that target BCL-2 family pro-survival proteins to induce tumour cell apoptosis represent a new era in cancer therapy. Clinical trials of navitoclax (ABT-263, which targets BCL-2, BCL-X L and BCL-W) have shown great promise, but encountered dose-limiting thrombocytopenia. Recent work has demonstrated that this is due to the inhibition of BCL-X L , which is essential for platelet survival. These findings raise new questions about the established model of platelet shedding by megakaryocytes, which is thought to be an apoptotic process. Here we generate mice with megakaryocyte-specific deletions of the essential mediators of extrinsic (Caspase-8) and intrinsic (BAK/BAX) apoptosis. We show that megakaryocytes possess a Fas ligand-inducible extrinsic apoptosis pathway. However, Fas activation does not stimulate platelet production, rather, it triggers Caspase-8-mediated killing. Combined loss of Caspase-8/BAK/BAX does not impair thrombopoiesis, but can protect megakaryocytes from death in mice infected with lymphocytic choriomeningitis virus. Thus, apoptosis is dispensable for platelet biogenesis. Platelets are anucleate blood cells essential for haemostasis and wound healing. They also play roles in inflammation, immunity, development of the lymphatic vasculature, and tumour metastases [1] . Platelets are produced by megakaryocytes, polyploid cells that develop primarily in the bone marrow (BM) and spleen. Megakaryocytes generate platelets by extruding cytoplasmic structures called proplatelets into the circulation [2] . These filamentous processes are sheared off to become preplatelets, which undergo maturation and fission to produce individual platelets. Over the last 15 years, a body of evidence has emerged to suggest that megakaryocytes deliberately undergo apoptosis in order to promote proplatelet formation and platelet shedding [3] . There are two distinct, convergent, pathways to apoptosis in mammals—the intrinsic and extrinsic—and both have been implicated in thrombopoiesis [4] . The intrinsic pathway is controlled by the BCL-2 family of proteins, which comprises three subsets: (1) the pro-survivals (BCL-2, BCL-X L (BCL2L1), BCL-W, MCL-1 and A1), (2) the multi-domain killers (BAK and BAX) and (3) the ‘BH3-only’ death initiators (for example, BIM, BID) [4] . In a healthy cell, the pro-survival proteins restrain BAK and BAX to prevent their activation. Pro-apoptotic signals (for example, DNA damage) cause induction of the BH3-only proteins, which overwhelm pro-survival activity and directly activate BAK/BAX. Active BAK/BAX induce mitochondrial outer membrane permeabilization (MOMP). The latter step is the ‘point of no return’, and triggers the efflux of apoptogenic factors, including Cytochrome c , from mitochondria. Together with apoptotic protease-activating factor 1 (APAF-1), Cytochrome c facilitates the activation of Caspase-9, leading to the proteolytic activation of the ‘effector’ caspases, Caspase-3 and Caspase-7, which cleave a multitude of protein substrates to effect cellular demolition. Beginning with the observation that mice overexpressing BCL-2 (ref. 5) [5] , or deficient in BIM [6] exhibit thrombocytopenia, several studies have suggested that the intrinsic pathway is required for thrombopoiesis. In cultured megakaryocytes, overexpression of BCL-X L [7] or treatment with the pan-caspase inhibitor z-VAD.fmk [8] , [9] was reported to reduce proplatelet formation. Conversely, in a human family with thrombocytopenia, premature platelet release into the BM was ascribed to the expression of a variant form of Cytochrome c with enhanced pro-apoptotic activity [10] . These observations suggest a critical, cell autonomous, role for the intrinsic pathway in platelet biogenesis. However, they are difficult to reconcile with evidence that pathophysiological insults trigger the apoptotic death of megakaryocytes, thereby causing thrombocytopenia. Traditional chemotherapeutic agents are a prime example [11] . Megakaryocyte apoptosis has also been implicated in a range of infection-related thrombocytopenias, including those associated with arenaviruses [12] , HIV [13] , dengue [14] and anthrax [15] . Apoptosis is also thought to contribute to thrombocytopenia in myelodysplastic syndrome [16] , and in immune-mediated thrombocytopenia [17] . Recent work utilizing genetically modified mice and pharmacological inhibitors of BCL-2 pro-survival proteins—the so-called ‘BH3 mimetics’—has established that both megakaryocytes and platelets contain a functional BAK/BAX-mediated intrinsic apoptosis pathway. In platelets, BCL-X L is the primary pro-survival protein that restrains BAK and BAX [18] , [19] , [20] , [21] . Accordingly, mutations in murine BCL-X L cause dose-dependent, cell-intrinsic reductions in platelet lifespan [18] , [19] , [22] . Moreover, pharmacological blockade of BCL-X L with the BH3 mimetic drugs ABT-737 (ref. 23) [23] or navitoclax (ABT-263) [24] triggers BAK/BAX-mediated platelet apoptosis [19] , [20] , [21] and thrombocytopenia in mice [19] , [25] dogs [21] and humans [26] . Indeed, the major dose-limiting toxicity of navitoclax in clinical trials has proven to be thrombocytopenia [26] . In contrast, ABT-199, a BCL-2-specific BH3 mimetic, shows potent anti-tumour activity in patients with chronic lymphocytic leukaemia, but has no significant effect on platelet counts [27] . In megakaryocytes, MCL-1 and BCL-X L are both required to keep BAK and BAX in check [18] , [28] , [29] . Their simultaneous deletion leads to a failure of megakaryopoiesis, haemorrhage and embryonic lethality. Accordingly, treatment of adult mice carrying a megakaryocyte-specific deletion of Mcl1 with ABT-737 (to block BCL-X L ) causes ablation of the megakaryocyte compartment. These effects are prevented by combined deletion of BAK/BAX. Importantly, while loss of BAK/BAX protects megakaryocytes from apoptotic stimuli (ABT-737 and others, for example, etoposide and carboplatin), it has no impact on thrombopoiesis at steady state or under conditions of stress [18] , [30] . Thus, the intrinsic apoptosis pathway is dispensable for platelet production. Rather than utilize it for platelet shedding, megakaryocytes must actively restrain the pathway in order to survive. This raises the question of what role the other apoptotic pathway—the extrinsic—plays in megakaryocytes and platelets. The extrinsic pathway is triggered by ligands binding to death receptors belonging to the tumour necrosis factor (TNF) receptor family, for example, Fas or TNF receptor-1 (ref. 4) [4] . This leads to activation of Caspase-8, the essential mediator of the pathway. Activated Caspase-8 can directly proteolytically activate Caspase-3/7, and also recruit the intrinsic apoptotic pathway via the BH3-only protein BID. Seminal work by Clarke et al. [8] suggested that activation of the extrinsic pathway in the cultured MEG-01 cell line or primary murine megakaryocytes—by treatment with Fas ligand (FasL) or agonistic Fas antibodies—augmented the production of platelet-like particles. This effect was specific to FasL, since TNF treatment did not increase particle yield. Moreover, delivery of a recombinant active form of Caspase-8 to cultured megakaryocytes doubled the number of cells that formed proplatelets. Similar results were obtained in explant cultures of human bone cores, which produced more platelet-like particles when incubated with agonistic Fas antibodies, and fewer when treated with the broad-spectrum caspase inhibitor, z-VAD.fmk. These data established the notion that activation of the extrinsic pathway promotes platelet shedding. Studies of the TNF-related apoptosis-inducing ligand (TRAIL), another death receptor ligand, have provided support for this model, suggesting that TRAIL can promote megakaryocyte maturation [31] , and that reductions in megakaryocyte apoptosis caused by decreased TRAIL expression might contribute to impaired thrombopoiesis in immune thrombocytopenia patients [32] . In the current study, we have generated mice with a megakaryocyte-specific deletion of Caspase-8 to examine the role of the extrinsic apoptosis pathway in megakaryocytes and platelets. In addition, using animals lacking both BAK and BAX, we have explored the extent of functional redundancy between the extrinsic and intrinsic apoptotic pathways in the megakaryocyte lineage, both at steady state, and in response to viral infection. We find that megakaryocytes, but not platelets, contain a FasL-responsive Caspase-8-mediated extrinsic apoptosis pathway that is dispensable for platelet production. Megakaryocytes possess an extrinsic apoptosis pathway We first examined the protein expression of Caspase-8, BID, FADD and Fas in platelets and in mature megakaryocytes purified from cultures of foetal liver cells. Megakaryocytes and platelets from Fas lpr/lpr mice, which carry a loss-of-function mutation in Fas [33] , were included as negative controls for Fas expression. By western blotting, we could readily detect Caspase-8 ( Fig. 1a ), BID ( Fig. 1b ) and FADD ( Fig. 1c ) in lysates of wild-type platelets and megakaryocytes. Flow cytometric analyses using Fas antibodies revealed the presence of Fas on the surface of wild-type megakaryocytes, but not platelets ( Fig. 1d ). 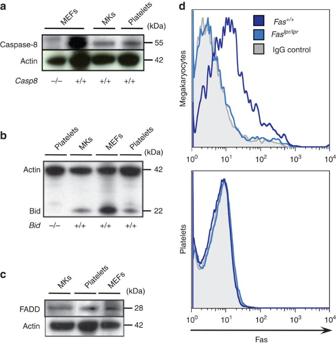Figure 1: Expression of extrinsic apoptosis pathway components in megakaryocytes and platelets. (a–c) Western blot analysis of protein lysates from platelets, foetal liver-derived megakaryocytes (MKs), and mouse embryonic fibroblasts (MEFs; control).Casp8−/−MEFs were used as a negative control for Caspase-8 andBid−/−platelets were used as a negative control for Bid protein. Probing for actin was used as a control for protein loading. (d) Fas surface expression was determined by flow cytometry on foetal liver-derived CD41+PI−live megakaryocytes and purified blood platelets. In addition to isotype control antibody staining, cells from Fas-deficientFaslpr/lprmice were used as a negative control. Figure 1: Expression of extrinsic apoptosis pathway components in megakaryocytes and platelets. ( a – c ) Western blot analysis of protein lysates from platelets, foetal liver-derived megakaryocytes (MKs), and mouse embryonic fibroblasts (MEFs; control). Casp8 −/− MEFs were used as a negative control for Caspase-8 and Bid −/− platelets were used as a negative control for Bid protein. Probing for actin was used as a control for protein loading. ( d ) Fas surface expression was determined by flow cytometry on foetal liver-derived CD41 + PI − live megakaryocytes and purified blood platelets. In addition to isotype control antibody staining, cells from Fas-deficient Fas lpr/lpr mice were used as a negative control. Full size image These observations suggested that while megakaryocytes and platelets express the cytoplasmic components of the extrinsic apoptosis pathway, only megakaryocytes are capable of responding to the classical extrinsic pathway agonist, FasL. We therefore tested the effect of FasL treatment on both cell types. Platelets purified from the peripheral blood of wild-type mice were incubated for 2 h at 37 °C with cross-linked FasL. Unlike thymocytes (used as a highly sensitive control cell population), we could not detect the active form of Caspase-8 in platelets exposed to FasL ( Fig. 2a ). Furthermore, unlike the BH3 mimetic compound ABT-737, which inhibits the essential platelet survival factor BCL-X L [18] , treatment of platelets with FasL did not trigger effector Caspase-3/7 activation ( Fig. 2b ), MOMP ( Fig. 2c ) or phosphatidylserine exposure ( Fig. 2d ). In contrast to platelets, mature BM- or foetal liver-derived wild-type megakaryocytes treated with FasL exhibited dose-dependent Caspase-8 activation, Caspase-3/7 activation and MOMP ( Fig. 3a–d ). The latter could be partially inhibited by co-incubation with the pan-caspase inhibitor Q-VD-OPh. Collectively, these data indicated that megakaryocytes, but not platelets, possess a functional extrinsic apoptosis pathway that can be activated by FasL. 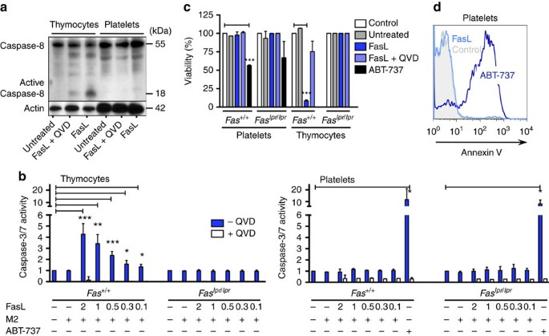Figure 2: FasL does not trigger apoptosis in platelets. (a) Western blot analysis of protein lysates from thymocytes and platelets for Caspase-8. Cells were treated with cross-linked FasL (2 μg ml−1) with or without inclusion of the pan-caspase inhibitor Q-VD-OPh (QVD) for 2 h at 37 °C. Probing for actin was used as control for protein loading. The uncropped blot is provided inSupplementary Fig. 6. (b) Effector Caspase-3/7 activity in platelets and thymocytes treated with cross-linked FasL (0.13–2 μg ml−1) or ABT-737 (1 μM) for 2 h at 37 °C, using the Caspase-Glo assay. Cells from Fas-deficientFaslpr/lprmice or co-treatment with QVD were used as negative controls. FasL was cross-linked by premixing Flag-tagged FasL with Flag mAb M2. Control indicates cells treated with M2 mAb only. Data represent fold increase compared with untreated cells.n=4 using wild-type (Fas+/+) cells; andn=3 usingFaslpr/lprcells. (c) ATP levels (viability) in platelets and thymocytes 4 h after treatment with FasL (2 μg ml−1) at 37 °C using the CellTiter-Glo assay. ABT-737 (1 μM) was a positive control. Cells from Fas-deficientFaslpr/lprmice were used as a negative control. Control indicates cells treated with Flag mAb M2 only and were set as 100% for cells of each genotype.n=3 separate experiments; ABT-737n=2. (d) Platelet phosphatidylserine exposure, as determined by Annexin V binding. Mouse platelets were treated with cross-linked FasL or ABT-737 (1 μM) for 2 h at 37 °C. Control indicates untreated. Data are presented as mean±s.d. Student’s unpairedt-test, *P<0.05; **P<0.005; ***P<0.001. Figure 2: FasL does not trigger apoptosis in platelets. ( a ) Western blot analysis of protein lysates from thymocytes and platelets for Caspase-8. Cells were treated with cross-linked FasL (2 μg ml −1 ) with or without inclusion of the pan-caspase inhibitor Q-VD-OPh (QVD) for 2 h at 37 °C. Probing for actin was used as control for protein loading. The uncropped blot is provided in Supplementary Fig. 6 . ( b ) Effector Caspase-3/7 activity in platelets and thymocytes treated with cross-linked FasL (0.13–2 μg ml −1 ) or ABT-737 (1 μM) for 2 h at 37 °C, using the Caspase-Glo assay. Cells from Fas-deficient Fas lpr/lpr mice or co-treatment with QVD were used as negative controls. FasL was cross-linked by premixing Flag-tagged FasL with Flag mAb M2. Control indicates cells treated with M2 mAb only. Data represent fold increase compared with untreated cells. n =4 using wild-type ( Fas +/+ ) cells; and n =3 using Fas lpr/lpr cells. ( c ) ATP levels (viability) in platelets and thymocytes 4 h after treatment with FasL (2 μg ml −1 ) at 37 °C using the CellTiter-Glo assay. ABT-737 (1 μM) was a positive control. Cells from Fas-deficient Fas lpr/lpr mice were used as a negative control. Control indicates cells treated with Flag mAb M2 only and were set as 100% for cells of each genotype. n =3 separate experiments; ABT-737 n =2. ( d ) Platelet phosphatidylserine exposure, as determined by Annexin V binding. Mouse platelets were treated with cross-linked FasL or ABT-737 (1 μM) for 2 h at 37 °C. Control indicates untreated. Data are presented as mean±s.d. Student’s unpaired t -test, * P <0.05; ** P <0.005; *** P <0.001. 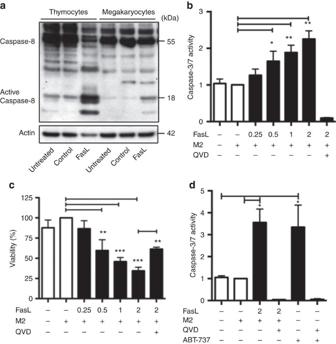Figure 3: FasL induces apoptosis in megakaryocytes. (a) Western blot analysis of protein lysates from BM-derived megakaryocytes and thymocytes for Caspase-8. Megakaryocytes were treated with cross-linked FasL (2 μg ml−1) for 5 h at 37 °C and thymocytes (1 μg ml−1) for 2 h. Control indicates cells treated with M2 mAb only. Probing for actin was used as control for protein loading. (b) Caspase 3/7 activity in foetal liver-derived megakaryocytes treated with FasL (0.25–2 μg ml−1) for 9 h at 37 °C. Caspase activity was measured using the Caspase-Glo assay. Co-treatment with the caspase inhibitor Q-VD-OPh (QVD) was used as a negative control. Data represent fold increase compared with control. Control indicates megakaryocytes treated with FLAG mAb M2 alone. (c) Mitochondrial function in foetal liver-derived megakaryocytes treated with FasL (0.25–2 μg ml−1) with or without inclusion of QVD. ATP levels in megakaryocytes were measured 48 h after treatment at 37 °C using the CellTiter-Glo assay. Control indicates megakaryocytes treated with FLAG mAb M2 alone and were set as 100%.n=3 separate experiments. Data represent mean±s.d. (d) Caspase-3/7 activity in BM-derived megakaryocytes treated with FasL (2 μg ml−1) for 9 h at 37 °C. QVD was used as a negative control, while ABT-737 was a positive control. Data represent fold increase compared with control (FLAG mAb M2 alone).n=2 separate experiments. One-way ANOVA with the Bonferroni multiple comparison test, *P<0.05; **P<0.005; ***P<0.001. Full size image Figure 3: FasL induces apoptosis in megakaryocytes. ( a ) Western blot analysis of protein lysates from BM-derived megakaryocytes and thymocytes for Caspase-8. Megakaryocytes were treated with cross-linked FasL (2 μg ml −1 ) for 5 h at 37 °C and thymocytes (1 μg ml −1 ) for 2 h. Control indicates cells treated with M2 mAb only. Probing for actin was used as control for protein loading. ( b ) Caspase 3/7 activity in foetal liver-derived megakaryocytes treated with FasL (0.25–2 μg ml −1 ) for 9 h at 37 °C. Caspase activity was measured using the Caspase-Glo assay. Co-treatment with the caspase inhibitor Q-VD-OPh (QVD) was used as a negative control. Data represent fold increase compared with control. Control indicates megakaryocytes treated with FLAG mAb M2 alone. ( c ) Mitochondrial function in foetal liver-derived megakaryocytes treated with FasL (0.25–2 μg ml −1 ) with or without inclusion of QVD. ATP levels in megakaryocytes were measured 48 h after treatment at 37 °C using the CellTiter-Glo assay. Control indicates megakaryocytes treated with FLAG mAb M2 alone and were set as 100%. n =3 separate experiments. Data represent mean±s.d. ( d ) Caspase-3/7 activity in BM-derived megakaryocytes treated with FasL (2 μg ml −1 ) for 9 h at 37 °C. QVD was used as a negative control, while ABT-737 was a positive control. Data represent fold increase compared with control (FLAG mAb M2 alone). n =2 separate experiments. One-way ANOVA with the Bonferroni multiple comparison test, * P <0.05; ** P <0.005; *** P <0.001. Full size image Caspase-8 is dispensable for platelet production To establish the requirement for the extrinsic pathway in megakaryocyte development and platelet production, we conditionally deleted Caspase-8 from the megakaryocyte lineage in vivo . For this, mice harbouring a floxed allele of Casp8 (ref. 34 ) were crossed with Pf4-Cre transgenic animals in which Cre recombinase is expressed under the control of the Platelet factor 4 promoter [35] . At weaning, Casp8 Pf4Δ/Pf4Δ mice were present at the expected Mendelian ratios and developed normally. Adult Casp8 Pf4Δ/Pf4Δ mice were healthy and fertile. Western blot analysis confirmed that Caspase-8 was efficiently deleted from megakaryocytes and platelets of these animals ( Fig. 4a ). Platelet counts and platelet survival curves in Casp8 Pf4Δ/Pf4Δ and Casp8 fl/fl littermate control mice were indistinguishable ( Fig. 4b,c ). Under resting conditions, surface expression of the platelet receptors GPIX, GPIbα, GPVI and CD41 was normal ( Supplementary Fig. 1A ). Moreover, Casp8 flfl and Casp8 Pf4Δ/Pf4Δ platelets stimulated with the single agonists PAR4-AP, convulxin or ADP exhibited similar levels of P-selectin surface exposure and CD41/61 integrin activation ( Supplementary Fig. 1B,C ). Caspase-8-deficient platelets treated with dual agonists (thrombin and convulxin) or the apoptotic stimulus ABT-737 exposed membrane phosphatidylserine at a level equivalent to wild type, indicating that, at least in vitro , Caspase-8 is not required for platelet pro-coagulant function ( Supplementary Fig. 1D ). 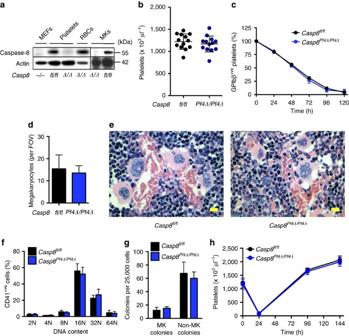Figure 4: Loss of Caspase-8 does not affect platelet production. (a) Western blot analysis of protein lysates from platelets, red blood cells (RBCs) and foetal liver-derived megakaryocytes (MKs). Δ/Δ indicatesPf4Cre-specific deletion. Negative control for Caspase-8 wasCasp8−/−mouse embryonic fibroblast (MEF) lysate. Probing for actin was used as a control for protein loading. (b) Platelet counts inCasp8Pf4Δ/Pf4Δmice andCasp8fl/flcontrol mice at 7 weeks of age. Each symbol represents an individual mouse. (c) Platelet survival curves inCasp8Pf4Δ/Pf4ΔandCasp8fl/flcontrol mice.n=5 mice per genotype. (d) Morphologically recognizable megakaryocytes in H&E-stained sections of BM fromCasp8Pf4Δ/Pf4ΔandCasp8fl/flcontrol micen=6Casp8fl/fl;n=8Casp8Pf4Δ/Pf4mice. (e) Representative images of H&E-stained sternum sections fromCasp8Pf4Δ/Pf4ΔandCasp8fl/flcontrol mice. Scale bar, 20 μm. Images were acquired on a Nikon Eclipse E600 microscope equipped with AxioCam MRc5 (Zeiss) and AxioVision 4.8. Scale bars were inserted with ImageJ 1.42q. (f) Ploidy distribution profile of CD41+BM cells inCasp8Pf4Δ/Pf4ΔandCasp8fl/flmice, as determined by flow cytometry.n=5 mice per genotype. (g) Haematopoietic colony forming units inCasp8Pf4Δ/Pf4ΔandCasp8fl/fladult mice. In total, 25,000 BM cells were cultured with SCF, IL-3 and erythropoietin in semisolid agar for 7 days. Non-megakaryocyte colonies represent the total of blast, granulocyte/macrophage, macrophage and eosinophil colonies.n=3 mice per genotype. (h) Platelet counts in mice treated with APS.n=6–13 mice per genotype. Data are presented as mean±s.d. Figure 4: Loss of Caspase-8 does not affect platelet production. ( a ) Western blot analysis of protein lysates from platelets, red blood cells (RBCs) and foetal liver-derived megakaryocytes (MKs). Δ/Δ indicates Pf4 Cre-specific deletion. Negative control for Caspase-8 was Casp8 −/− mouse embryonic fibroblast (MEF) lysate. Probing for actin was used as a control for protein loading. ( b ) Platelet counts in Casp8 Pf4Δ/Pf4Δ mice and Casp8 fl/fl control mice at 7 weeks of age. Each symbol represents an individual mouse. ( c ) Platelet survival curves in Casp8 Pf4Δ/Pf4Δ and Casp8 fl/fl control mice. n =5 mice per genotype. ( d ) Morphologically recognizable megakaryocytes in H&E-stained sections of BM from Casp8 Pf4Δ/Pf4Δ and Casp8 fl/fl control mice n =6 Casp8 fl/fl ; n =8 Casp8 Pf4Δ/Pf4 mice. ( e ) Representative images of H&E-stained sternum sections from Casp8 Pf4Δ/Pf4Δ and Casp8 fl/fl control mice. Scale bar, 20 μm. Images were acquired on a Nikon Eclipse E600 microscope equipped with AxioCam MRc5 (Zeiss) and AxioVision 4.8. Scale bars were inserted with ImageJ 1.42q. ( f ) Ploidy distribution profile of CD41 + BM cells in Casp8 Pf4Δ/Pf4Δ and Casp8 fl/fl mice, as determined by flow cytometry. n =5 mice per genotype. ( g ) Haematopoietic colony forming units in Casp8 Pf4Δ/Pf4Δ and Casp8 fl/fl adult mice. In total, 25,000 BM cells were cultured with SCF, IL-3 and erythropoietin in semisolid agar for 7 days. Non-megakaryocyte colonies represent the total of blast, granulocyte/macrophage, macrophage and eosinophil colonies. n =3 mice per genotype. ( h ) Platelet counts in mice treated with APS. n =6–13 mice per genotype. Data are presented as mean±s.d. Full size image Megakaryocyte numbers, morphology and ploidy in Casp8 Pf4Δ/Pf4Δ mice were comparable to those in Casp8 fl/fl littermates ( Fig. 4d–f ), and enumeration of megakaryocyte progenitors in semisolid agar cultures revealed no differences ( Fig. 4g ). These results indicated that Caspase-8 is dispensable for platelet biogenesis. To rule out the possibility that this is true only at steady state, we tested the ability of Casp8 fl/fl and Casp8 Pf4Δ/Pf4Δ mice to recover from acute thrombocytopenia induced by injection of anti-platelet serum (APS). Twenty-four hours after a single dose of APS, platelet counts had fallen to almost undetectable levels in mice of both genotypes ( Fig. 4h ). Subsequently, Casp8 fl/fl and Casp8 Pf4Δ/Pf4Δ animals mounted a robust recovery of similar magnitude and kinetics, with platelet counts exceeding baseline by 6 days post-APS injection. Together, these data demonstrate that Caspase-8 is dispensable for normal megakaryopoiesis, platelet production and platelet lifespan. FasL triggers Caspase-8-mediated apoptosis in megakaryocytes To understand more fully the biochemical pathway downstream of Fas activation in megakaryocytes, we examined the effect of FasL treatment on megakaryocytes lacking components of the extrinsic or intrinsic apoptotic pathways. Mature megakaryocytes were gradient-purified from cultures of wild-type, Fas lpr/lpr , Casp8 Pf4Δ/Pf4Δ or Bak −/− Bax −/− foetal liver cells, and then treated with FasL. Viability and proplatelet formation were subsequently tracked over 3 days. In agreement with the data presented in Fig. 3 , we found that wild-type megakaryocytes were readily killed by treatment with FasL ( Fig. 5a ), and that this was accompanied by a dose-dependent failure of proplatelet formation ( Fig. 5b , Supplementary Table 1 ). Instead of elaborating proplatelets, FasL-treated wild-type cells exhibited membrane blebbing ( Supplementary Fig. 2 ). Conversely, the viability of Fas lpr/lpr and Casp8 Pf4Δ/Pf4Δ megakaryocytes, and their ability to form proplatelets, was unaffected by FasL treatment ( Fig. 5a,b ). Thus, activation of the extrinsic apoptosis pathway by FasL results in Caspase-8-mediated megakaryocyte death. Co-incubation with the pan-caspase inhibitor Q-VD-OPh did not rescue proplatelet formation in wild-type megakaryocytes. Given the resistance of Casp8 Pf4Δ/Pf4Δ megakaryocytes to FasL treatment, this suggests that, despite the demonstrated ability of Q-VD-OPh to inhibit Caspase-8 (ref. 36) [36] , at the dose employed it did not reduce Caspase-8 activity sufficiently to allow proplatelet formation to proceed. Furthermore, loss of BAK and BAX also failed to protect FasL-treated megakaryocytes against Caspase-3/7 activation, or rescue viability and proplatelet formation ( Fig. 5c ) indicating that megakaryocytes are Type I cells with regard to the extrinsic apoptosis pathway, that is, the apoptotic signal mediated by Caspase-8 does not require amplification through BID-mediated engagement of the intrinsic apoptosis pathway to induce cell death [37] , [38] . 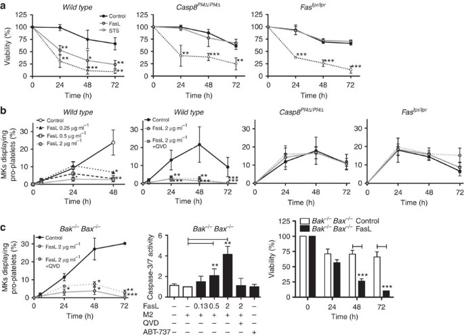Figure 5: FasL induces the apoptotic death of megakaryocytes. (a) Effects of FasL on megakaryocyte viability, as assessed by trypan blue staining. E13.5 foetal liver cells were cultured in serum free media in TPO for 3 days. On day 4, gradient purified megakaryocytes from wild-type,Faslpr/lprandCasp8Pf4Δ/Pf4Δmice were treated with cross-linked FasL (2 μg ml−1), staurosporine (STS, 10 μM) or left untreated (control). Megakaryocytes negative for trypan blue as assessed by light microscopy were classed as viable cells.n=3 independent experiments per genotype. (b) Proplatelet formation by cultured megakaryocytes. E13.5 foetal liver cells were cultured in SFM in TPO for 3 days. On day 4, large megakaryocytes were purified from a BSA gradient and reseeded (time 0) to investigate proplatelet formation after treatment with cross-linked FasL with or without the pan-caspase inhibitor Q-VD-OPh (QVD). Control indicates megakaryocytes treated with FLAG mAb M2 only. Percentage of proplatelet-forming megakaryocytes (MKs) per day compared with time 0.n=4–8 wild-type, except for FasL 0.25 μg ml−lwheren=2;n=4Faslpr/lpr;n=4Casp8Pf4Δ/Pf4Δbiological replicates. Absolute numbers are presented inSupplementary Table 1. (c) Proplatelet formation, Caspase-3/7 activity and viability in foetal liver-derivedBak−/−Bax−/−megakaryocytes. Proplatelet formation was performed as described inb. Caspase activity was assessed after treatment with FasL (0.13–2 μg ml−1) for 5 h at 37 °C. Co-treatment with QVD or treatment with ABT-737 was used as controls. Data represent fold increase compared with control (FLAG mAb M2 alone). Viability measured by CellTiter-Glo assay inBak−/−Bax−/−megakaryocytes treated with FasL (2 μg ml−1) up to 72 h. Control indicates megakaryocytes treated with FLAG mAb M2 alone.n=2–3 biological replicates. Data represent mean±s.d. Student’s unpairedt-test, *P<0.05; **P<0.005; ***P<0.001. Figure 5: FasL induces the apoptotic death of megakaryocytes. ( a ) Effects of FasL on megakaryocyte viability, as assessed by trypan blue staining. E13.5 foetal liver cells were cultured in serum free media in TPO for 3 days. On day 4, gradient purified megakaryocytes from wild-type, Fas lpr/lpr and Casp8 Pf4Δ/Pf4Δ mice were treated with cross-linked FasL (2 μg ml −1 ), staurosporine (STS, 10 μM) or left untreated (control). Megakaryocytes negative for trypan blue as assessed by light microscopy were classed as viable cells. n =3 independent experiments per genotype. ( b ) Proplatelet formation by cultured megakaryocytes. E13.5 foetal liver cells were cultured in SFM in TPO for 3 days. On day 4, large megakaryocytes were purified from a BSA gradient and reseeded (time 0) to investigate proplatelet formation after treatment with cross-linked FasL with or without the pan-caspase inhibitor Q-VD-OPh (QVD). Control indicates megakaryocytes treated with FLAG mAb M2 only. Percentage of proplatelet-forming megakaryocytes (MKs) per day compared with time 0. n =4–8 wild-type, except for FasL 0.25 μg ml −l where n =2; n =4 Fas lpr/lpr ; n =4 Casp8 Pf4Δ/Pf4Δ biological replicates. Absolute numbers are presented in Supplementary Table 1 . ( c ) Proplatelet formation, Caspase-3/7 activity and viability in foetal liver-derived Bak −/− Bax −/− megakaryocytes. Proplatelet formation was performed as described in b . Caspase activity was assessed after treatment with FasL (0.13–2 μg ml −1 ) for 5 h at 37 °C. Co-treatment with QVD or treatment with ABT-737 was used as controls. Data represent fold increase compared with control (FLAG mAb M2 alone). Viability measured by CellTiter-Glo assay in Bak −/− Bax −/− megakaryocytes treated with FasL (2 μg ml −1 ) up to 72 h. Control indicates megakaryocytes treated with FLAG mAb M2 alone. n =2–3 biological replicates. Data represent mean±s.d. Student’s unpaired t -test, * P <0.05; ** P <0.005; *** P <0.001. Full size image Response of the megakaryocytic lineage to FasL in vivo Our results demonstrated that in megakaryocytes, FasL induces Caspase-8-mediated (but BAX/BAK-independent) apoptotic death, concomitant with a failure of proplatelet formation. While this is consistent with the well-characterized role of FasL and Fas in other cell types, it runs counter to the notion that activation of the extrinsic pathway facilitates platelet shedding by megakaryocytes [8] . We therefore tested the effect of Fas activation in vivo . Injection of FasL or agonistic Fas antibodies into wild-type mice results in massive hepatocellular apoptosis and death of the animals within hours of treatment [39] . To circumvent this, we generated BM chimaeras. Fas lpr/lpr CD45.2 mice were lethally irradiated and reconstituted with wild-type CD45.1 GFP +ve or Casp8 Pf4Δ/Pf4Δ CD45.2 BM. In recipients of wild-type cells, at 8 weeks post-transplantation, 99±2% of peripheral blood platelets (CD41 +ve GFP +ve ) and 85±5% of lymphocytes (CD45.1 +ve GFP +ve ) were donor-derived. In recipients of Casp8 Pf4Δ/Pf4Δ BM, we determined donor contribution to the megakaryocyte lineage by western blotting for Caspase-8 in platelet lysates from individual mice ( Supplementary Fig. 3 ). After quantifying by densitometry scanning, animals exhibiting a 77±4% reduction in platelet Caspase-8 levels were included in the study. 9.5 weeks post-transplantation, chimaeric mice were injected intravenously with 0.25 μg g −1 body weight FasL cross-linked with 2 μg mouse FLAG mAb per μg of FasL. Control mice were injected with FLAG mAb alone. Wild-type mice treated with FasL became sick within 3 h. Analysis of a group of these animals collected 2.5 h post-FasL treatment revealed severe liver damage, with obvious signs of haemorrhage and many condensed, fragmented cell nuclei present ( Fig. 6a ). These mice were anaemic ( Supplementary Fig. 4 ) and severely thrombocytopenic ( Fig. 6b ), although BM megakaryocyte numbers and morphology were normal ( Fig. 6a,c ). 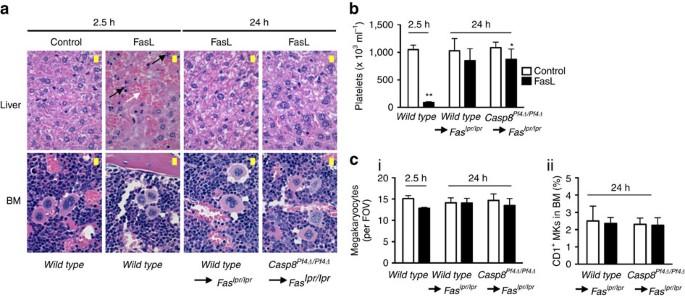Figure 6: FasL treatment does not increase platelet countsin vivo. (a) Liver and BM histology from wild-type mice and BM chimaeras treated with FasL.Faslpr/lprmice reconstituted with wild-type CD45.1GFP+BM (wild-type→Faslpr/lpr),Faslpr/lprmice reconstituted withCasp8Pf4Δ/Pf4ΔBM (Casp8Pf4Δ/Pf4Δ→Faslpr/lpr) and wild-type mice were injected i.v. with 0.25 μg g−1body weight of recombinant FasL aggregated with 2 μg FLAG (M2) mAb per μg FasL or, as a control, with FLAG mAb M2 alone. Wild-type mice were culled 2.5 h after injection, BM reconstitutedFaslpr/lprmice at 24 h. Black arrows indicate condensed fragmented nuclei and white arrows point to haemorrhage observed in the livers of treated wild-type mice. Scale bar, 20 μm. Images were acquired on a Nikon Eclipse E600 microscope equipped with AxioCam MRc5 (Zeiss) and AxioVision 4.8. Scale bars were inserted with ImageJ 1.42q. (b) Platelet counts in mice described ina. Severe thrombocytopenia was observed after 2.5 h in FasL injected wild-type mice. Data represent mean±s.d.n=5–6 wild-type→Faslpr/lpr;n=6Casp8Pf4Δ/Pf4Δ→Faslpr/lprandn=2 wild-type mice per group. (c) (i) Megakaryocyte counts in H&E-stained sections of BM. Data represent mean per field of view (FOV; × 200) from 10 fields per individual mouse. (ii) Percent CD41+megakaryocytes (MKs) in BM assessed by flow cytometry. Data represent mean±s.d.n=5–6 wild-type→Faslpr/lpr;n=6Casp8Pf4Δ/Pf4Δ→Faslpr/lprandn=2 wild-type mice per group. Student’s unpairedt-test, **P<0.005. Figure 6: FasL treatment does not increase platelet counts in vivo . ( a ) Liver and BM histology from wild-type mice and BM chimaeras treated with FasL. Fas lpr/lpr mice reconstituted with wild-type CD45.1GFP + BM (wild-type→ Fas lpr/lpr ), Fas lpr/lpr mice reconstituted with Casp8 Pf4Δ/Pf4Δ BM ( Casp8 Pf4Δ/Pf4Δ → Fas lpr/lpr ) and wild-type mice were injected i.v. with 0.25 μg g −1 body weight of recombinant FasL aggregated with 2 μg FLAG (M2) mAb per μg FasL or, as a control, with FLAG mAb M2 alone. Wild-type mice were culled 2.5 h after injection, BM reconstituted Fas lpr/lpr mice at 24 h. Black arrows indicate condensed fragmented nuclei and white arrows point to haemorrhage observed in the livers of treated wild-type mice. Scale bar, 20 μm. Images were acquired on a Nikon Eclipse E600 microscope equipped with AxioCam MRc5 (Zeiss) and AxioVision 4.8. Scale bars were inserted with ImageJ 1.42q. ( b ) Platelet counts in mice described in a . Severe thrombocytopenia was observed after 2.5 h in FasL injected wild-type mice. Data represent mean±s.d. n =5–6 wild-type→ Fas lpr/lpr ; n =6 Casp8 Pf4Δ/Pf4Δ → Fas lpr/lpr and n =2 wild-type mice per group. ( c ) (i) Megakaryocyte counts in H&E-stained sections of BM. Data represent mean per field of view (FOV; × 200) from 10 fields per individual mouse. (ii) Percent CD41 + megakaryocytes (MKs) in BM assessed by flow cytometry. Data represent mean±s.d. n =5–6 wild-type→ Fas lpr/lpr ; n =6 Casp8 Pf4Δ/Pf4Δ → Fas lpr/lpr and n =2 wild-type mice per group. Student’s unpaired t -test, ** P <0.005. Full size image In contrast to their wild-type counterparts, all the Fas lpr/lpr BM chimaeras were alive 24 h post-FasL injection, at which point they were taken for analysis. As anticipated, both Fas lpr/lpr :wild-type and Fas lpr/lpr : Casp8 Pf4Δ/Pf4Δ chimaeras exhibited normal liver morphology ( Fig. 6a ). Peripheral blood erythrocyte and leukocyte numbers were unchanged, although trends towards monocytopenia and eosinophilia were observed in both groups of chimaeric mice ( Supplementary Fig. 4 ). Platelet counts in Fas lpr/lpr :wild-type animals were mildly reduced ( Fig. 6b ), but the difference was not statistically significant. A similar trend was apparent in Fas lpr/lpr : Casp8 Pf4Δ/Pf4Δ chimaeras, indicating that the modest drop in platelet counts was not due to activation of the extrinsic apoptosis pathway in platelets. BM megakaryocyte numbers and morphology were also normal in the aforementioned FasL-injected chimaeras ( Fig. 6a,c ). Collectively, these data indicate that acute FasL-induced thrombocytopenia in mice is not caused by the direct action of FasL on BM-derived cells, and that FasL treatment in vivo does not stimulate platelet production in the short term. Platelet production proceeds independently of apoptosis The BAK/BAX-mediated intrinsic apoptosis pathway is dispensable for platelet production [18] . Our results indicated that loss of the extrinsic pathway alone also has no major deleterious effects on platelet biogenesis. To examine any potential functional redundancy between these two apoptotic pathways, we elected to simultaneously disable both, by generating mice with megakaryocyte-specific deletions of Casp8 and Bax, and a constitutive deletion of Bak . Casp8 fl/fl Pf4Cre + animals were crossed with Bak − / − Bax fl/fl mice to generate the triple knockout and relevant control littermates. Mice of all genotypic classes were born at the expected Mendelian ratios and were outwardly healthy and fertile. Western blotting of platelet lysates confirmed efficient deletion of BAK, BAX and Caspase-8 in the megakaryocyte lineage ( Supplementary Fig. 5A ). Upon examination, we found that Bak −/− Bax Pf4Δ/Pf4Δ Casp8 Pf4Δ/Pf4Δ triple knockout mice were phenotypically similar to their Bak −/− Bax Pf4Δ/Pf4Δ counterparts, exhibiting no impairment of platelet production. The number, morphology and ploidy of mature megakaryocytes in the BM of Bak −/− Bax Pf4Δ/Pf4Δ and Bak −/− Bax Pf4Δ/Pf4Δ Casp8 Pf4Δ/Pf4Δ animals were equivalent to those of wild-type mice ( Fig. 7a , Supplementary Fig. 5B ). Serum thrombopoietin (TPO) levels were modestly elevated in Bak −/− Bax Pf4Δ/Pf4Δ Casp8 Pf4Δ/Pf4Δ animals ( Supplementary Fig. 5C ). Consistent with previous reports, a significant number of what appeared to be naked megakaryocyte nuclei were seen in the BM of Bak −/− Bax Pf4Δ/Pf4Δ mice [18] , and this phenomenon was also observed in Bak −/− Bax Pf4Δ/Pf4Δ Casp8 Pf4Δ/Pf4Δ triple knockout animals ( Fig. 7a ). As in Bak −/− Bax Pf4Δ/Pf4Δ mice, platelet lifespan and platelet counts were significantly elevated in Bak −/− Bax Pf4Δ/Pf4Δ Casp8 Pf4Δ/Pf4Δ triple knockout animals ( Fig. 7b,c ), an effect attributable to loss of BAK, the critical regulator of platelet lifespan at steady state [19] . Bak −/− Bax Pf4Δ/Pf4Δ Casp8 Pf4Δ/Pf4Δ mice mounted a wild-type response to experimentally induced thrombocytopenia ( Fig. 7d ). Thus, the combined functions of BAK, BAX and Caspase-8 are dispensable for platelet production, demonstrating that there is no physiological requirement for activation of either the intrinsic or extrinsic apoptosis pathways in thrombopoiesis. 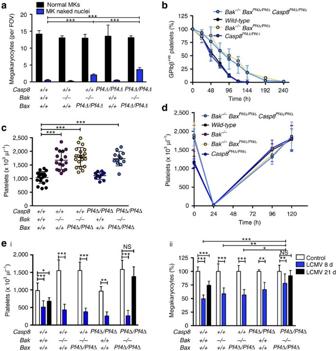Figure 7: Platelet production occurs independently of the intrinsic and extrinsic apoptosis pathways. (a) Morphologically recognizable megakaryocytes (MKs) and megakaryocytic naked nuclei in H&E-stained sections of BM from wild-type (WT),Bak−/−,Bak−/−BaxPf4Δ/Pf4,Casp8Pf4Δ/Pf4andBak−/−BaxPf4Δ/Pf4Casp8Pf4Δ/Pf4Δmice. Mean per field of view (FOV; × 200) from 10 fields per individual mouse;n=6 WT;n=10Bak−/−;n=3Bak−/−BaxPf4Δ/Pf4;n=8Casp8Pf4Δ/Pf4andn=4Bak−/−BaxPf4Δ/Pf4Casp8Pf4Δ/Pf4Δmice. (b) Platelet survival curves in WT,Bak−/−BaxPf4Δ/Pf4,Casp8Pf4Δ/Pf4ΔandBak−/−BaxPf4Δ/Pf4Casp8Pf4Δ/Pf4Δmice. Platelets were labelled via i.v. injection of a DyLight 488-conjugated anti-GPIbβ Ab.n=3–4 mice per genotype. (c) Blood platelet counts in wild-type (WT),Bak−/−,Bak−/−BaxPf4Δ/Pf4, Casp8Pf4Δ/Pf4ΔandBak−/−BaxPf4Δ/Pf4Casp8Pf4Δ/Pf4Δmice at 7–10 weeks of age. Each symbol represents an individual mouse. (d) Platelet counts in mice treated with APS. Cohorts of mice were bled,n=6–14 (t=0 h);n=8–25 (t=24 h);n=5–12 (t=96 h);n=6–13 (t=120 h) mice per genotype, at the indicated time points. (e) (i) Blood platelet and BM (ii) megakaryocyte numbers 8 and 21 days after LCMV Docile infection in C57BL/6 mice. The infection dose was 2 × 106p.f.u. LCMV Docile per mouse. Megakaryocytes were scored per field of view in BM H&E stained sections. Megakaryocyte numbers in untreated control mice were set as 100%.n=4–18 WT;n=10–13;Bak−/−;n=4–6Bak−/−BaxPf4Δ/Pf4;n=4Casp8Pf4Δ/Pf4andn=4–11Bak−/−BaxPf4Δ/Pf4Casp8Pf4Δ/Pf4Δmice per group. Data are presented as mean±s.d. One-way ANOVA with the Bonferroni multiple comparison test (a,c), Student’s unpairedt-test (e), *P<0.05; **P<0.005; ***P<0.001. Figure 7: Platelet production occurs independently of the intrinsic and extrinsic apoptosis pathways. ( a ) Morphologically recognizable megakaryocytes (MKs) and megakaryocytic naked nuclei in H&E-stained sections of BM from wild-type (WT), Bak −/− , Bak −/− Bax Pf4Δ/Pf4 , Casp8 Pf4Δ/Pf4 and Bak −/− Bax Pf4Δ/Pf4 Casp8 Pf4Δ/Pf4Δ mice. Mean per field of view (FOV; × 200) from 10 fields per individual mouse; n =6 WT; n =10 Bak −/− ; n =3 Bak −/− Bax Pf4Δ/Pf4 ; n =8 Casp8 Pf4Δ/Pf4 and n =4 Bak −/− Bax Pf4Δ/Pf4 Casp8 Pf4Δ/Pf4Δ mice. ( b ) Platelet survival curves in WT, Bak −/− Bax Pf4Δ/Pf4 , Casp8 Pf4Δ/Pf4Δ and Bak −/− Bax Pf4Δ/Pf4 Casp8 Pf4Δ/Pf4Δ mice. Platelets were labelled via i.v. injection of a DyLight 488-conjugated anti-GPIbβ Ab. n =3–4 mice per genotype. ( c ) Blood platelet counts in wild-type (WT), Bak −/− , Bak −/− Bax Pf4Δ/Pf4 , Casp8 Pf4Δ/Pf4Δ and Bak −/− Bax Pf4Δ/Pf4 Casp8 Pf4Δ/Pf4Δ mice at 7–10 weeks of age. Each symbol represents an individual mouse. ( d ) Platelet counts in mice treated with APS. Cohorts of mice were bled, n =6–14 ( t =0 h); n =8–25 ( t =24 h); n =5–12 ( t =96 h); n =6–13 ( t =120 h) mice per genotype, at the indicated time points. ( e ) (i) Blood platelet and BM (ii) megakaryocyte numbers 8 and 21 days after LCMV Docile infection in C57BL/6 mice. The infection dose was 2 × 10 6 p.f.u. LCMV Docile per mouse. Megakaryocytes were scored per field of view in BM H&E stained sections. Megakaryocyte numbers in untreated control mice were set as 100%. n =4–18 WT; n =10–13; Bak −/− ; n =4–6 Bak −/− Bax Pf4Δ/Pf4 ; n =4 Casp8 Pf4Δ/Pf4 and n =4–11 Bak −/− Bax Pf4Δ/Pf4 Casp8 Pf4Δ/Pf4Δ mice per group. Data are presented as mean±s.d. One-way ANOVA with the Bonferroni multiple comparison test ( a , c ), Student’s unpaired t -test ( e ), * P <0.05; ** P <0.005; *** P <0.001. Full size image We next considered the possibility that, although BAK/BAX-mediated intrinsic apoptosis signalling and the Caspase-8-dependent extrinsic apoptosis pathway are not required by megakaryocytes for platelet production, other components of these pathways might play a role. This could conceivably involve their activation via a non-canonical apoptotic signalling pathway, or, alternatively, be the result of them having non-cell death-associated functions, such as have been ascribed to the effector caspases, Caspase-3 and -7 (refs 40 , 41 , 42 ). We therefore generated BM chimaeras by lethally irradiating adult C57BL/6 mice and reconstituting them with foetal liver cells from animals lacking both Caspase-3 (ref. 43) [43] and Caspase-7 (ref. 44) [44] , mice deficient for APAF-1 (ref. 45) [45] , or mice homozygous for a mutation in Cytochrome c that diminishes its binding to APAF-1 (ref. 46) [46] . Eight to ten weeks post-transplantation, efficient engraftment of the hosts was confirmed by flow cytometric analysis, and platelet counts were measured. No statistically significant differences were observed between the various groups of recipient mice (wild-type 1,037±253 × 10 3 μl −1 , n =12 recipients; Casp3 −/− Casp7 −/− 992±204 × 10 3 μl −1 , n =5; Apaf1 −/− 899±132 × 10 3 μl −1 , n =10; Cycs tm1Mak/tm1Mak 1,002±172 × 10 3 μl −1 , n =11), demonstrating that these apoptotic regulators are dispensable for platelet biogenesis at steady state. Megakaryocyte apoptosis in a viral infection model It has previously been demonstrated that cultured Bak −/− Bax −/− megakaryocytes show resistance to diverse apoptotic stimuli, such as ABT-737 and etoposide, and that combined loss of BAK and BAX from the haematopoietic system significantly ameliorates carboplatin-induced thrombocytopenia in mice [18] . We hypothesized that megakaryocytes lacking both the intrinsic and extrinsic pathways would be protected in other pathophysiological stress conditions that have been suggested to cause their apoptotic death, such as viral infection [13] , [47] , [48] . We therefore examined the impact on the megakaryocyte compartment of lymphocytic choriomeningitis virus (LCMV). Infection of mice with the LCMV Docile is a well-established model of chronic viremia that bears similarities with HIV and hepatitis B and C infections in humans [49] . After 8 days of infection with LCMV Docile, a point at which mice exhibit high viral titers and mild hepatitis [50] , experimental cohorts were taken for analysis. Consistent with previous studies employing the LCMV variant WE [51] , [52] , which causes an acute viral infection, a significant drop in circulating platelet counts was observed in wild-type mice relative to uninfected controls ( Fig. 7e(i)) . This was accompanied by a significant reduction in the number of BM megakaryocytes ( Fig. 7e(ii) ). While blockade of the intrinsic (BAK/BAX loss) or extrinsic (Caspase-8 loss) pathway, or both, did not ameliorate LCMV-induced thrombocytopenia at day 8, it did protect megakaryocytes, which, in infected Bak −/− Bax Pf4Δ/Pf4Δ Casp8 Pf4Δ/Pf4Δ triple knockout mice, were present at ~78% of pre-infection numbers (compared with 50% in wild-type counterparts). During the chronic phase (that is, 21 days after infection) when platelet and megakaryocyte levels were significantly reduced in wild-type mice, they were almost normal in Bak −/− Bax Pf4Δ/Pf4Δ Casp8 Pf4Δ/Pf4Δ triple knockout mice ( Fig. 7e(i,ii)) . These data indicate that in mice infected with LCMV Docile, megakaryocytes undergo apoptosis. We have shown that megakaryocytes possess a functional, canonical extrinsic apoptosis pathway, which can be activated by FasL. The activation of this pathway by FasL does not stimulate platelet production, in contrast to what has been previously suggested [8] , rather, it leads to Caspase-8-mediated megakaryocyte killing with consequent failure of proplatelet formation. Disabling the pathway by deleting Caspase-8 in megakaryocytes had no impact on megakaryocyte and platelet numbers in vivo , either at steady state or in response to thrombopoietic stress. Remarkably, additional deletion of BAK and BAX, the essential mediators of the intrinsic apoptosis pathway [53] , did not result in any impairment of platelet production. Thus, the combined functions of the intrinsic and extrinsic apoptosis pathways—as currently defined—are dispensable for thrombopoiesis ( Fig. 8 ). 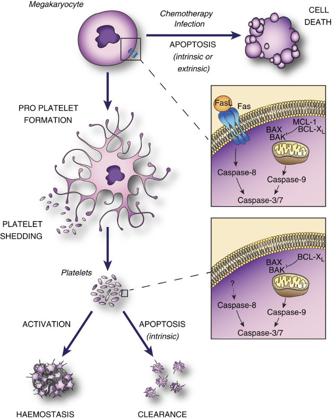Figure 8: The role of apoptosis in megakaryocyte and platelet biology. Megakaryocytes possess functional BAK/BAX-mediated intrinsic, and FasL-inducible extrinsic apoptosis pathways. Both pathways must be restrained during megakaryocyte growth and development in order to allow platelet production to occur. The apoptotic pathways can be triggered in response to chemotherapy or infection. Once shed into the circulation, platelet lifespan is regulated by the intrinsic apoptosis pathway. Platelets lack the Fas receptor, and the role of Caspase-8 and the extrinsic pathway in platelets is yet to be established. Figure 8: The role of apoptosis in megakaryocyte and platelet biology. Megakaryocytes possess functional BAK/BAX-mediated intrinsic, and FasL-inducible extrinsic apoptosis pathways. Both pathways must be restrained during megakaryocyte growth and development in order to allow platelet production to occur. The apoptotic pathways can be triggered in response to chemotherapy or infection. Once shed into the circulation, platelet lifespan is regulated by the intrinsic apoptosis pathway. Platelets lack the Fas receptor, and the role of Caspase-8 and the extrinsic pathway in platelets is yet to be established. Full size image Some of the differences between our results and those of Clarke et al. [8] might potentially be explained by the choice of reagents, particularly the use of megakaryocytic cell lines and the fluoromethylketone caspase inhibitor z-VAD.fmk. The latter is known to have a range of non-caspase targets including calpains and cathepsins and to exert non-specific toxicity [54] . Accordingly, we have shown previously that while z-VAD.fmk impairs proplatelet formation by cultured mouse megakaryocytes, the more specific difluorophenoxymethylketone-based caspase inhibitor Q-VD-OPh does not [18] , [36] . In addition, for the majority of assays described in the Clarke study, Fas ligation was performed using agonistic Fas antibody (which does not always perfectly mimic FasL), rather than the more potent aggregated FasL [55] . The results of our BM chimaera experiments were somewhat inconclusive. Platelet and megakaryocyte numbers in Fas lpr/lpr mice reconstituted with wild-type BM remained stable when the animals were injected with FasL. This clearly demonstrates that the severe, rapid onset thrombocytopenia induced by FasL in unmanipulated wild-type mice is not caused by the direct killing of megakaryocytes, nor platelets (consistent with the lack of Fas expression on the platelet surface), but is the result of FasL-induced damage to non-haematopoietic tissues, most likely the liver. What the experiment did not provide is definitive evidence that FasL is either pro- or anti-thrombopoietic in vivo . The simplest explanation is a technical failure to achieve sufficient concentrations of FasL in the haematopoietic microenvironment. Indeed, if FasL was truly capable of promoting platelet production in vivo , that would be the only conceivable explanation for why platelet counts did not rise in Fas lpr/lpr :wild-type chimaeras. However, given the rapid and profound response to FasL treatment observed in unmanipulated wild-type control mice, this seems unlikely. We believe a more plausible scenario is that megakaryocytes in vivo are exposed to a range of survival promoting factors (for example, fibroblast growth factor-4, stromal-derived factor-1, Interleukin (IL)-6, IL-11, and stem cell factor (SCF)) that render them less susceptible to FasL-induced killing compared with when they are placed in tissue culture. This is supported by previous work demonstrating that wild-type megakaryocytes are sensitive to ABT-737 in vitro but not in vivo [18] . It remained formally possible that, rather than full-blown apoptosis driven by BAK, BAX and/or Caspase-8, megakaryocytes undergo a more limited or specialized apoptosis-like process, mediated by the downstream apoptotic machinery, and activated independently of BAK, BAX and Caspase-8. However, our results show that mice with a haematopoietic system lacking APAF-1, the apoptosis-inducing function of Cytochrome c , or the apoptotic effector Caspases 3/7, exhibit normal platelet counts. Together with prior work demonstrating that Caspase-9, the apoptotic initiator caspase, is not required for platelet production at steady state [56] , the now overwhelming weight of evidence indicates that the apoptotic cascade is dispensable for platelet biogenesis. Our findings stand in stark contrast with studies suggesting that megakaryocytes deliberately undergo apoptosis in order to facilitate platelet shedding [5] , [6] , [7] , [8] , [9] , [10] , [48] . One explanation for the discrepancy might be that megakaryocytes have evolved their own unique apoptotic pathways, which utilize effectors other than BAK, BAX and Caspase-8. This seems unlikely, given that apoptotic stimuli, such as ABT-737, etoposide or FasL can efficiently trigger megakaryocyte death, which can be blocked by deletion of BAK/BAX and/or Caspase-8, respectively. It is true that in cultured megakaryocytes, the effects of staurosporine, a widely used inducer of the intrinsic apoptosis pathway in other cell types, cannot be ameliorated by loss of BAK and BAX [18] , nor Caspase-8 ( Fig. 5a ). This may be consistent with the existence of alternative cell death pathways in megakaryocytes. However, staurosporine does not stimulate thrombopoiesis, rather, it causes mitochondrial damage, failure of proplatelet formation and death. Taken together, our results and those of several recent studies [18] , [22] , [28] , [29] , [30] , [56] , [57] leave little room for the notion that apoptosis, as it is currently defined [54] , is required for, or can augment, platelet production by megakaryocytes. It remains possible that one or more components of the apoptotic machinery may play a role in the process, but convincing evidence for this has yet to emerge. One criticism that can be made of our current work is that it has been conducted entirely in mice or primary cells derived from them. Do human megakaryocytes behave differently to their murine equivalent? While this possibility cannot be formally excluded, the major apoptotic pathways are highly conserved [4] . The most instructive example of this in relation to the megakaryocyte lineage has been the clinical development of the BH3 mimetic anti-cancer drugs. These agents are specifically designed to inhibit BCL-2 family pro-survival proteins. Navitoclax (ABT-263), one of the first BH3 mimetics to enter clinical trials, targets BCL-XL, BCL-2 and BCL-W [24] . Since the initial discovery that BCL-XL is the critical factor responsible for regulating murine platelet survival and lifespan [19] , it has been shown that Navitoclax, or its relative ABT-737 (ref. 23) [23] , trigger platelet apoptosis and consequent thrombocytopenia not only in mice [19] , [25] , but also in dogs [21] and humans [20] , [21] , [26] . Caspase inhibitors can block the short-term apoptotic effects of navitoclax and ABT-737 in human platelets [20] , [21] , just as they do in mouse [56] . These and other data suggest that the human megakaryocyte lineage possesses apoptotic pathways that are similar (if not identical) in nature to their murine counterparts. The extent to which activation or dysregulation of apoptotic pathways contributes to megakaryocyte and platelet abnormalities in the context of human disease remains to be fully elucidated. In mice infected with LCMV Docile, genetic deletion of Casp8 , Bak and Bax had no impact on the severity of thrombocytopenia during the acute phase (day 8). In contrast, in chronic phase (day 21) when platelet counts in wild-type mice were still significantly below baseline, they had already recovered in Bak −/− Bax Pf4Δ/Pf4Δ Casp8 Pf4Δ/Pf4Δ triple knockout mice. Thus, the acute thrombocytopenia induced by LCMV is not caused by the apoptotic death of platelets. This is not to say that platelets in mice suffering an acute LCMV infection do not undergo apoptosis, merely that some other mechanism underlies their sequestration and/or clearance from the circulation. Whether there are settings in which platelet apoptosis induced by an infectious agent does contribute to thrombocytopenia is yet to be established, but there is evidence to support the idea. Platelets from dengue virus-infected patients exhibit increased signs of apoptosis [58] , as do platelets exposed to Helicobacter pylori in vitro [59] . Perhaps most compelling is recent work demonstrating that Escherichia coli and Staphylococcus aureus isolates from sepsis patients induce features of apoptosis in platelets in vitro , including the calpain-mediated degradation of BCL-X L [60] . The fact that pathogenic bacteria can target the key platelet pro-survival protein certainly lends weight to the notion that aberrant platelet apoptosis might contribute to infection-induced thrombocytopenia. Unlike platelets, megakaryocyte numbers at day 8 were increased in Bak −/− Bax Pf4Δ/Pf4Δ Casp8 Pf4Δ/Pf4Δ animals relative to wild-type controls, indicating that during the acute phase of an LCMV infection, a significant proportion of megakaryocytes undergo apoptosis. This also appeared to be the case during chronic phase, where, at day 21, megakaryocyte numbers were reduced in wild-type mice, but had returned to pre-infection levels in Bak −/− Bax Pf4Δ/Pf4Δ Casp8 Pf4Δ/Pf4Δ animals. Thus, combined ablation of the intrinsic and extrinsic apoptosis pathways can protect the megakaryocyte compartment in LCMV-infected mice. The mechanism or mechanisms that trigger megakaryocyte apoptosis in this setting remain to be established. Previous work by Binder et al. [51] has shown that in mice infected with the LCMV-WE clone, deletion of the interferon-α/β receptor (IFNAR) prevented the ~50% decrease in megakaryocyte counts observed 3 days post infection. Paradoxically, megakaryocytes in IFNAR −/− animals showed a dramatic increase in positivity for LCMV-specific antigen. The latter might reflect the fact that (a) loss of IFNAR-mediated signalling protects megakaryocytes from virally induced death, but renders them more susceptible to viral infection, or (b) IFNAR status has no bearing on infection, but the amelioration of cell death means infected megakaryocytes are more readily detected. Regardless, our data together with the Binder study suggest that elevated type I interferon levels contribute to the apoptotic death of megakaryocytes in vivo . Interferons have been known to negatively impact the megakaryocyte lineage for more than 30 years [61] . Their clinical use is associated with thrombocytopenia, and a host of studies have demonstrated that they can inhibit megakaryopoiesis in vivo and in vitro . Several mechanisms have been proposed, including the suppression of progenitor cell proliferation [61] , as well as inhibition of cytoplasmic maturation and platelet production, but there is no published evidence to suggest that interferons induce megakaryocyte apoptosis directly. Interferons have been linked to the induction of apoptosis in tumour cells; this is primarily thought to be the result of transcriptionally mediated changes in the levels of pro-apoptotic factors such as Caspase-8 (ref. 61) [61] . Similarly, a recent study demonstrated that type I interferons produced as a consequence of Toll-like receptor stimulation kill dendritic cells via upregulation of the BH3-only proteins Bim, Puma and/or Noxa [12] . Perhaps, in the context of a viral infection, high levels of type I interferons in vivo sensitize megakaryocytes to apoptotic death via a related mechanism. Given their pleiotropic nature, however, it seems likely that type I interferons also affect megakaryocytes indirectly, and this is supported by work involving Junín virus, the cause of Argentine haemorrhagic fever [62] . Studies utilizing mice carrying a megakaryocyte-specific deletion of IFNAR will be required to resolve the cell intrinsic versus cell extrinsic effects of type I interferons on the megakaryocyte lineage. Animals Bak [53] , Bax [63] , Apaf1 −/− (ref. 45 ), Casp3 −/− (ref. 43 ) and Casp7 −/− (ref. 44 ) knockout, Cycs tm1Mak/tm1Mak knockin [46] , Casp8 and Bax floxed [64] , [65] , Fas lpr/lpr [66] , Pf4-Cre [35] and UBC-GFP [67] transgenic mice have been previously described. All mutations had been backcrossed onto the C57BL/6 background for at least 10 generations prior to this study. All animal experiments complied with the regulatory standards of, and were approved by, the Walter and Eliza Hall Institute Animal Ethics Committee. Materials Dimethylsulphoxide, thrombin, A23187, ADP, PAR4-AP, propidium iodide, staurosporine and cross-linking anti-FLAG mAb (M2) were from Sigma-Aldrich. ABT-737 was provided by Abbvie. Q-VD-OPh, FLAG-tagged human recombinant soluble FasL and convulxin were from Enzo Life Sciences. The enhanced chemiluminescence system was from Millipore, the protease inhibitor cocktail, Complete, was from Roche, 4–12% Bis-Tris gels (NuPAGE) were from Invitrogen and calibration beads 3.5–4.0 μm were from Spherotech Inc. Antibodies used for immunoblotting included: rat anti-mouse Caspase-8 (clones 3B10, IG12, 1:1,000) and rat anti-mouse FADD (clone 7A2, 1:2,500) were obtained from Enzo Life Sciences; rat anti-mouse BID (clone 2DI, 1:1,000) [37] was a gift from D. Huang, The Walter & Eliza Hall Institute (WEHI); rabbit polyclonal anti-BAK (1:2,000) was from Sigma-Aldrich; rabbit polyclonal anti-BAX (1:1,000) from Millipore; anti-actin-HRP from Santa Cruz; and goat anti-rat IgG-HRP from Southern Biotech. Antibodies used for flow cytometry included: X488, fluorescently conjugated-GPIbα (Xia.G5, 1:100), -GPIX (Xia.B4, 1:100), -GPVI (JAQ1, 1:100), -P-selectin (Wug.E9, 1:100) and activated β3-integrin (JON/A, 1:100) were obtained from Emfret Analytics GmbH and Co. KG; FITC-, PE- or APC-conjugated anti-mouse, CD41 (MWReg30, 1:100), CD45.1 (A20, 1:200), CD45.2 (1:200), CD45R/B220 (RA3-6B2, 1:200), biotinylated anti-mouse Fas (Jo2, 1:50) and fluorescently conjugated streptavidin and Annexin V were purchased from BD Biosciences. Haematology Automated cell counts were performed on blood collected by cardiac puncture or from the retro-orbital plexus into Microtainer tubes containing EDTA (Sarstedt), using an Advia 2120 haematological analyzer (Siemens). Megakaryocytes were counted manually in sections of sternum and spleen stained with haematoxylin and eosin (H&E) with a minimum of 10 high-power fields ( × 200) analysed. Haematopoietic progenitors were cultured with SCF, IL-3 and erythropoietin in semisolid agar for 7 days as described [18] . Acute thrombocytopenia was induced by i.v. injection of 100 μl of Cedarlane’s APS (per 20 g mouse) at a 1:25 pre-dilution. This reduces platelet counts to near undetectable levels within 24 h, followed by rebound thrombocytosis [9] . Primary megakaryocyte culture Foetal livers were removed at embryonic day (E) 13.5 and transferred into Dulbecco’s modified Eagle’s (DME) medium (high glucose version) with 10% foetal calf serum (FCS) (Gibco, Paisley, UK). BM was harvested from murine bones and flushed into DME medium with 2% FCS. The cells were lineage depleted by incubation with a mix of biotinylated antibodies (CD4, CD2, CD3, CD5, CD8, Ter119, B220, CD19, Gr-1, Ly6G, F4/F8, CD127; WEHI) in KDS BSS 2% FCS, followed by anti-biotin magnetic microbeads (Myltenyi Biotec, NSW, Australia) and MAC LS columns (Myltenyi Biotec). Single cell suspensions were cultured for 3–5 days at 5 × 10 5 cells per ml in serum-free medium (SFM) [68] supplemented with 100 ng ml −1 murine TPO (WEHI) at 37 °C, 5% CO 2 and mature megakaryocytes purified using a discontinuous BSA density gradient (3, 1.5 and 0%). Cells were harvested in the 3% layer after 35 min [69] . Proplatelet formation assay Large foetal liver-derived megakaryocytes were seeded in 96-well plates at a concentration of 100–300 cells/well into SFM with 100 ng ml −1 TPO [69] . Cells were cultured at 37 °C with 5% CO 2 with or without the addition of FLAG-tagged aggregated FasL (2 μg ml −1 ) and/or Q-VD-OPh (50 μM). 1 × FLAG-tagged FasL (0.25–2 μg ml −1 ) was aggregated with 10 × FLAG mAb (2.5–20 μg ml −1 ). The M2 FLAG mAb control group received 20 μg ml −1 . Megakaryocytes were examined by light microscopy and the percentage of megakaryocytes displaying proplatelets was calculated by dividing by the total number of cells at start. Megakaryocyte ploidy and receptor expression BM was harvested from femurs of 8–10 week-old mice into 1 ml of CATCH medium and megakaryocyte ploidy was studied by staining with CD41-FITC mAb and propidium iodide and data acquired by flow cytometry (LSR II, BD) [8] . Fas surface expression was determined by flow cytometry on foetal liver-derived CD41 +ve PI −ve megakaryocytes. Serum TPO Serum TPO levels were measured using the mouse TPO Quantikine ELISA (R&D Systems) according to the manufacturer’s instructions. Caspase activity and cell viability assays Purified platelets (suspended at 5 × 10 8 cells per ml in buffer B), thymocytes (10 7 cells per ml in DME medium with 10% FCS) and BSA gradient-purified megakaryocytes (3 × 10 4 cells per ml in SFM with TPO) were seeded into 96-well plates and then incubated at 37 °C, 5% CO 2 with or without the addition of FLAG-tagged aggregated FasL, Q-VD-OPh (50 μM) or ABT-737 (1–5 μM). 1 × FLAG-tagged FasL (0.25–2 μg ml −1 ) was aggregated with 10 × FLAG mAb (2.5–20 μg ml −1 ). The control group was treated with FLAG mAb at 20 μg ml −1 . Caspase-Glo 3/7 reagents (Promega) were added to thymocytes and platelets after 2 h and to megakaryocytes after 9 h of treatment. The luminescence of each sample was determined in a plate-reading LumiSTAR Galaxy luminometer (BMG Labtech). Alternatively, CellTiter Glo reagents (Promega) were added after 4 h to thymocytes and platelets and after 48 h to megakaryocytes to determine cell viability by measuring ATP levels. Cell death was also assessed by seeding megakaryocytes (2 × 10 3 cells per ml) harvested from BSA gradients in SFM with TPO with or without the addition of cross-linked FasL (2 μg ml −1 ). At 24 h time points, cell viability was assessed by light microscopy after the addition of trypan blue 0.4% (Gibco). Video microscopy Megakaryocytes were generated from BM as detailed in the primary megakaryocyte culture and transferred to optically transparent ibiTreat tissue culture-treated sterile μ-slide 8-well (Ibidi) plates. Experiments were performed on a Live Cell Observer with a fully motorized Axiovert 200 inverted microscope (Carl Zeiss, Inc.) driven by the Axiovision 4.7 software (Carl Zeiss, Inc.). Cells were maintained on the stage within a humidified chamber at 37 °C and 5% CO 2 . Time-lapse images were acquired every 10 min for 21 h, with an AxioCam MRm camera (Carl Zeiss, Inc.) using a × 20/0.8 objective. Mitotracker Red FM 50 nM (Molecular Probes), DAPI 0.1 μg ml −1 and FLAG-tagged FasL 1 μg ml −1 aggregated with FLAG mAb 10 μg ml −1 were added 1 h before commencing time-lapse images. Representative still images were prepared in ImageJ. Platelet preparation and activation Murine blood was obtained by cardiac puncture into 0.1 volume of Aster-Jandl anticoagulant (85 mM sodium citrate, 69 mM citric acid and 20 mg ml −1 glucose, pH 4.6) [69] . Platelet-rich plasma was obtained by centrifugation at 125 g for 8 min, followed by centrifugation of the supernatant buffy coat at 125 g for 8 min. Platelets were washed by two sequential centrifugations at 860 g for 5 min in 140 mM NaCl, 5 mM KCl, 12 mM trisodium citrate, 10 mM glucose and 12.5 mM sucrose, pH 6.0 (buffer A). The platelet pellet was resuspended in 10 mM Hepes, 140 mM NaCl, 3 mM KCl, 0.5 mM MgCl 2 , 10 mM glucose and 0.5 mM NaHCO 3 , pH 7.4 (buffer B) and platelets resuspended in buffer B at a concentration of 1–5 × 10 8 cells per ml and counted by flow cytometric analysis by adding a known concentration of FACS calibration beads (Spherotech). To determine the surface expression of platelet receptors, purified platelets were stained with fluorescently conjugated antibodies to GPIbα, GPIX, GPVI or CD41 for 20 min in buffer B at room temperature (RT) and samples were further diluted and directly examined by flow cytometry (FACSCalibur, BD). When biotinylated mouse Fas specific mAb (Jo2) was used, a secondary incubation with streptavidin-FITC for 40 min at RT was performed, including an additional wash (buffer A) by centrifugation (5 min, 860 g, RT) prior to analysis. In platelet activation experiments, purified platelets were treated with or without the single agonists ADP (6.25–50 μM), Convulxin (12.5–50 ng ml −1 ), PAR4-AP (30–250 μM) for 20 min at RT in the presence of CaCl 2 (1 mM) and activation of the β3 integrin (JON/A) or P-selectin exposure were assessed by flow cytometry. To determine platelet exposure of phosphatidylserine in response to thrombin plus convulxin (Thr 0.5–1 U ml −1 ; Cvx 50–100 ng ml −1 , 10 min RT), ionophore A23187 (1 μM, 10 min), cross-linked FasL (2 μg ml −1 , 2 h at 37 °C) or the intrinsic apoptosis inducer ABT-737 (0.06–0.5 μM, 90 min 37 °C), treated platelets were incubated for 20 min at RT with Annexin V and CD41-APC mAb in Annexin V buffer (Invitrogen) before flow cytometric analysis. Reticulated platelets were enumerated by thiazole orange staining. Thiazole orange powder was dissolved in methanol at 1 mg ml −1 then pre-diluted at 1:10,000 in PBS. To label platelets, CD41-APC was diluted 1:50 in PBS. Sample was prepared by mixing 1 μl of blood (in EDTA) with 9 μl CD41-APC and 50 μl of diluted thiazole in PBS. Sample was incubated for 20 min at RT, fixed with 1% PFA in PBS and analysed on a FACSCalibur [9] . Platelet turnover studies 7-10 week-old male and female mice were injected i.v. with 0.15 μg g −1 body weight of X488 (Emfret, Germany), a rat-derived IgG against the platelet GPIbβ receptor and platelet lifespan was measured by flow cytometry [69] . Mice were bled from tail vein every 24 or 48 h and platelets were identified in platelet-rich plasma as being CD41 +ve and the proportion of X488 +ve platelets remaining at each time point was assessed. SDS–PAGE and western blot analysis Platelets were lysed in NP40 lysis buffer and megakaryocytes, thymocytes, erythrocytes and MEFs were lysed in RIPA buffer. Proteins were separated on 4–12% Bis-Tris gels (NuPAGE; Invitrogen) under reducing conditions, transferred onto Immobilon-P membranes (Micron Separation) and immunoblotted with various Abs, followed by incubation with secondary HRP-conjugated Abs and enhanced chemiluminescence. BM chimaeras Fas lpr/lpr male and female mice, in which the haematopoietic system was reconstituted at the age of 7 weeks with GFP-positive (CD45.1) male 19-week-old wild-type BM or BM extracted from male 17-week-old Casp8 Pf4Δ/Pf4Δ (CD45.2) mice, were generated after lethal irradiation (2 × 5.5 Gy spaced by 2 h) and injection of 4 × 10 6 BM cells. Donor cell contribution was tested 8 weeks after transplantation by determining the proportions of GFP +ve platelets (CD41 +ve ) and lymphocytes (CD45.1 +ve , CD45R/B220) in peripheral blood. Caspase-8 protein levels in platelets were examined by western blotting, and quantified by densitometry. Apaf-1 −/− , Cycs tm1Mak/tm1Mak , Casp3 −/− Casp7 −/− BM chimaeras were generated by transplantation of 2 × 10 6 E13.5 foetal liver cells (C57BL/6 CD45.2 + ) into lethally irradiated male congenic CD45.1 + recipients. Treatment of mice with FasL BM reconstituted Fas lpr/lpr mice (9.5 weeks post transplant, 16.5 week-old male and female mice) and wild-type control mice were injected into the tail vein with 0.25 μg g −1 body weight human recombinant FLAG-tagged FasL cross-linked with 2 μg FLAG mAb per μg FasL [37] . Wild-type mice were culled after 2.5 h and BM chimaeras after 24 h. Infection of mice with LCMV All mice were kept in a specific pathogen-free environment until infected, at which time animals were moved to a quarantine room. Infection was initiated by injecting 2 × 10 6 PFU LCMV Docile into the tail vein of 7–9 week-old mice. Blood and organs were collected 8 or 21 days after infection. Virus was propagated on L929 cells [70] . Statistical analyses Statistical significance between two treatment groups was analysed using an unpaired Student’s t- test with two-tailed P values. One-way ANOVA with the Bonferroni multiple comparison test was applied where appropriate (GraphPad Prism Software Version 6.0b). * P <0.05; ** P <0.005; *** P <0.001 or as otherwise stated. Data are presented as mean±s.d. How to cite this article: Josefsson, E. C. et al. Platelet production proceeds independently of the intrinsic and extrinsic apoptosis pathways. Nat. Commun. 5:3455 doi: 10.1038/ncomms4455 (2014).